A borane laser Emission from electronically excited species forms the basis for an important class of light sources—lasers. So far, commercially available solution-processed blue-emitting laser materials are based on organic compounds or semiconductor nanocrystals that have significant limitations: either low solubility, low chemical- and/or photo-stability and/or uncompetitive prices. Here we report a novel and competitive alternative to these existing laser materials that is based on boron hydrides, inorganic cluster compounds with a rich and diverse chemistry. We demonstrate that solutions of the borane anti -B 18 H 22 show, under pulsed excitation, blue laser emission at 406 nm with an efficiency (ratio of output/input energies) of 9.5%, and a photostability superior to many of the commercially available state-of-the-art blue laser dyes. This demonstration opens the doors for the development of a whole new class of laser materials based on a previously untapped resource for laser technology—the boranes. Few devices have extended the frontiers of science and technology to the same degree that lasers have, leading to a global market in lasers worth billions of US dollars annually [1] . Blue-emitting lasers are tools of uppermost importance to many applications, ranging from spectroscopy and material processing to underwater communications, biotechnology and medicine [2] , [3] . After nearly 55 years of intense research and development on laser technology, researchers are still pursuing cost-effective solution-processed gain materials for direct generation—as opposed to frequency conversion processes—of tunable, efficient and photostable laser emission in the blue spectral region. Until now, both the commercial availability of this kind of laser media [4] , [5] , [6] , [7] and most of the aligned research activity have been directed to the development of either organic-based materials, such as laser dyes [8] , conjugated polymers [9] and oligomers [10] , or inorganic-based colloidal quantum dots (QDs) [11] . Although highly efficient and tunable emission is readily available from these materials, there are still important drawbacks that limit widespread commercial usage, such as low solubility in common solvents and polymers, low chemical stability and/or photostability and/or lengthy and costly synthetic procedures. In this regard, organic–inorganic halide perovskites have recently emerged as an alternative and very promising solution-processed gain material. They exhibit a range of advantageous features such us high absorption coefficients, low emission thresholds, easy manipulation of emission wavelength by changing the perovskite stoichiometry and record-breaking photostabilities [12] . While having a huge potential, they are presently not commercially available and are intrinsically restricted to the solid state. Most problematic is the fact that stimulated emission at the blue spectral edge using these species is only achieved at 150 K, which is an important drawback compromising their applicability. In an attempt to overcome the above limitations, and to provide a radically new solution to the demand for blue laser materials, we have turned our attention to boranes (boron hydrides), a group of inorganic compounds previously unconsidered in laser technology. Boron has one valence electron fewer than its number of valence orbitals. This ostensible electron-deficiency necessitates hydrides of boron to share electron density in quasi-aromatic delocalized fashions [13] . It does this by forming molecules of polyhedral cluster geometries [14] . These geometries represent an architectural bridge in the structural continuum that stretches from the highly condensed clusters adopted by the late transitional metals to the open chains and ring formations found in the hydrocarbons. As chemical and physical behaviour is often a function of structure, then the boron hydrides have, with their unique polyhedral molecular geometries, large potential for novel properties. This is indeed the case, and in recent times boron hydrides—or boranes as these compounds are more commonly referred to—and their derivatives are proving promising candidates for application in medicinal fields [15] , microelectronics [16] , reversible capture of small molecules [17] , catalysis [18] , in the modification of surfaces [19] and as enhancers of the fluorescent properties of various luminescent organic polymers or fluorophores [20] . We have recently become interested in the photophysical properties of the binary borane anti -B 18 H 22 , the centrosymmetric isomer of octadecaborane(22) that has a polyhedral structure resembling a split soccer ball ( Fig. 1 ). Of all the known binary boranes (compounds consisting only of boron and hydrogen), anti -B 18 H 22 is the only one to have the property of fluorescence. This attribute was first noticed by Hawthorne et al. [21] , and yet only recently described comprehensively, including a full consideration of all transitions between ground and excited electronic states of the molecule [22] . In this latter study, anti -B 18 H 22 was revealed to exhibit an intense blue fluorescence at 407 nm ( Fig. 2a ) with a quantum yield approaching unity ( Φ F =0.97). This unexpectedly strong fluorescence arises from a population of a metastable excited state that has a lifetime of 11.2 ns [22] , which is easily long enough for ready participation in stimulated emission. These fundamental photophysical parameters suggest that anti -B 18 H 22 could make a good laser material, however, not all strongly fluorescent compounds can fulfil the stringent pumping and gain conditions required to achieve laser emission, and, despite its high quantum yield of fluorescence, anti -B 18 H 22 has a molar extinction coefficient (a measure of how strongly a chemical species absorbs light) ( Fig. 2a ) 10 times lower than those of commercial organic dyes with absorption/emission in the same spectral region. Therefore the question arises: will the photophysical advantages inherent to anti -B 18 H 22 , such as its high quantum yield of fluorescence and long excited-state lifetime, outweigh and overcome its associated limitations if operated as a laser? Thus, we embarked on a rigorous study of the laser performance of anti -B 18 H 22 and an evaluation of the potential of this compound as a laser material. 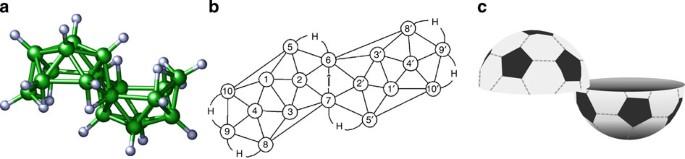Figure 1: The molecular structure ofanti-B18H22. (a) structure as defined by single-crystal X-ray diffraction45. (b) Aerial view showing numbering and connectivities. (c) Split football visual analogy. Figure 1: The molecular structure of anti -B 18 H 22 . ( a ) structure as defined by single-crystal X-ray diffraction [45] . ( b ) Aerial view showing numbering and connectivities. ( c ) Split football visual analogy. 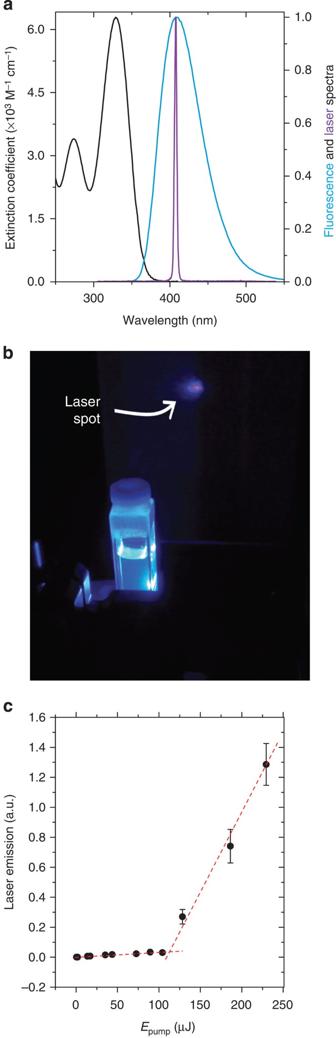Figure 2: Photophysical and laser properties ofanti-B18H22. (a) Molar extinction coefficient, fluorescence and laser spectra fromanti-B18H22. (b) Photograph of laser emission from a cyclohexane solution ofanti-B18H22. (c) Plot of laser output intensity versus pump energy for a 50 mM solution ofanti-B18H22. Error bars account for s.d. over 9 acquisitions. Full size image Figure 2: Photophysical and laser properties of anti -B 18 H 22 . ( a ) Molar extinction coefficient, fluorescence and laser spectra from anti -B 18 H 22 . ( b ) Photograph of laser emission from a cyclohexane solution of anti -B 18 H 22 . ( c ) Plot of laser output intensity versus pump energy for a 50 mM solution of anti -B 18 H 22 . Error bars account for s.d. over 9 acquisitions. Full size image Laser properties of anti -B 18 H 22 Remarkably, solutions of anti -B 18 H 22 indeed show broadband laser emission centred at 406 nm ( Fig. 2a ) and bright blue-purple laser spots ( Fig. 2b ) when pumped with a nitrogen laser ( λ =337.1 nm) at energies well above the laser threshold. A significant—and maximum—laser energy-conversion efficiency of 9.5% was measured using a 50 mM cyclohexane solution. The laser threshold of this sample, understood as the pump energy at which a change in the slope of the output intensity versus pump energy curve occurs, was found to be 115 μJ ( Fig. 2c ). Solutions with a concentration of 25 mM showed a slightly lower efficiency (8%), whereas the efficiency of 10 mM solutions could not be detected with the setup used, although a clear laser line and spot were observed. By contrast, samples of concentration 5 mM did not show laser emission at the maximum pump energy available, while concentrations higher than 50 mM could not be satisfactorily prepared due to diminishing solubility of the compound in cyclohexane. Nevertheless, it is noteworthy that such a high concentration is two orders of magnitude greater than that achievable with organic blue dyes, even despite the solvent being organic and the solute inorganic. This, in itself, is intriguing and indicative of the differences between the boranes and organic compounds. For purposes of experimental thoroughness, we employed two other standard pumping sources in addition to the nitrogen laser (see Alternative laser sources in the Methods section), but optimal laser efficiency was achieved with the latter. These results unambiguously demonstrate that anti -B 18 H 22 renders blue laser emission with a good laser efficiency (~10%). Encouragement may be taken in the consideration that the very first organic laser dyes rendered efficiencies of about 4% [23] , [24] . Furthermore, it must be emphasized that this is a new type of laser gain medium in that anti -B 18 H 22 is an inorganic molecular species with structural and chemical properties unlike those of conventional laser materials. In this regard, the boranes, with their wide emission bands and large Stoke’s shifts ( Fig. 2a ), could become an alternative to the present conjugated carbon-based laser dyes as the active medium for widely tunable high-power laser sources. Comparison with commercial dye laser diphenylstilbene To assess the prospects of anti -B 18 H 22 as a genuine alternative laser source, and to place our results into context, we compared them with data obtained using the same experimental setup for the commercial dye laser, Diphenylstilbene (DPS), which is a binary hydrocarbon of similar molecular size and has absorption and emission bands overlapping with those of anti -B 18 H 22 (see Supplementary Fig. 1 ). A 0.5 mM solution of DPS—pumped with the same nitrogen laser—gives laser emission at 408 nm, with an efficiency of 29% and a threshold of 15 μJ. On first consideration, it is quite surprising that anti -B 18 H 22 , a compound with a superior quantum yield of 0.97, renders laser efficiencies lower than DPS, an organic dye with a quantum yield of 0.74 (ref. 25 ). In an attempt to rationalize this unexpected efficiency deficiency in the borane compound, we employed a theoretical formalism developed by Heudorfer and Marowsky [26] . This formalism relates the laser threshold and efficiency with the spectroscopic properties of the emitter, as well as the cavity properties. Although this model is more suited for steady-state conditions (long-pulse or continuous-wave excitation), its results are still informative for short-pulse operation. Heudorfer and Marowsky [26] found that the threshold pump photon flux ( I pc ) can be expressed as: where κ and p are cavity-related parameters (see the Methods section for a full description), N tot is the ground-state population density, τ is the fluorescence lifetime, σ ap 0 and σ al 0 are the ground-state absorption cross-sections at the pump and laser wavelengths, σ e is the stimulated emission cross-section and σ al 1 is the excited singlet-state absorption cross-section at the laser wavelength. Terms for triplet-state effects have not been included in equation (1), as they are negligible under short-pulse excitation. In terms of energy, the laser threshold is expressed as: where h is Planck’s constant, ν p is the frequency of the pumping light, A is the pumping area and τ p is the pump-pulse width (see Supplementary Table 1 for values used in equations (1) and (2)). Assuming that, in a first approximation, excited-state absorption is negligible ( σ al 1 =0), the calculated laser threshold ( E th ) for DPS and its experimentally measured value are very similar (12 μJ (calc.) versus 15 μJ (exp.)). In comparison, the calculated and experimental values of E th for anti -B 18 H 22 differ substantially (1 μJ (calc.) versus 115 μJ (exp.)). As laser threshold and laser efficiency are related (the lower the threshold, the higher the laser efficiency), the two orders of magnitude difference between calculated and experimental values of E th for anti -B 18 H 22 suggest that there is yet scope for improvement in efficiency of this, the first, borane laser. The above equation (1) alludes to what factors are the probable causes for this loss in laser efficiency. A first consideration is a reduction in the fluorescence quantum yield due to self-quenching [27] (both static and dynamic) at the relatively high borane concentrations used in the laser solutions. This would reduce the fluorescence lifetime ( τ ) and, according to equation (1), increase the threshold. In fact, preliminary measurements suggest that the fluorescence quantum yield of anti -B 18 H 22 in highly concentrated cyclohexane solutions only marginally decreases to Φ F =0.86 (as measured with an integrating sphere for a 5 mM solution). A second consideration is that, at such high concentrations, there are solubility problems. Indeed, we have detected the presence of microcrystallites in solutions of higher concentration that cause a significant level of optical scattering ( α SC ~0.17 cm −1 ). A third consideration as a further plausible source of losses is the presence of excited-state absorption at the laser emission wavelength ( σ al 1 >0), although this effect cannot be easily proved. Finally, triplet–triplet and ground-state ( σ al 0 ) absorptions at the laser wavelength can be ruled out, as they were not detected in the previous work [22] . Interestingly, despite all these losses, anti -B 18 H 22 still emits blue laser light with an efficiency of nearly 10%. Encouragingly, if these effects could be, at least partially, mitigated, then anti -B 18 H 22 could in due course prove to be a laser of remarkable efficiency. Photostability of anti -B 18 H 22 In terms of commercial utility and feasibility of laser materials, efficiency is not the only crucial variable to be considered. A further important parameter is the photostability of the laser emission over long operation times. Ideally, a high resistance to active medium photodegradation under repeated pumping is sought after [28] . A reasonable evaluation of the photostability of individual laser materials can be obtained by irradiating a small amount of solution with exactly the same pumping energy and geometry as used for the laser experiments (see Methods for details), and monitoring the evolution of the laser-induced fluorescence (LIF) intensity with respect to the number of pump pulses (see Methods for details). The use of LIF to track the active medium photodegradation makes it possible to monitor how many active molecules have been degraded, as there is a linear relation between the excited molecules and LIF intensity. As such, we are able to determine an intrinsic photodegradation rate that enables absolute comparisons with different active media irrespective of the cavity configuration/parameters and sample concentrations used. Thus, for a 60 μl 5 mM solution of anti -B 18 H 22 , an absorbed energy dose of 25 kJ l −1 was needed to reduce the LIF intensity to 90% of its initial value ( Fig. 3 ). In terms of time, this means 20 min pumping at the maximum pump energy of 370 μJ at 15 Hz. In contrast, an absorbed energy dose of 25 kJ l −1 reduced the LIF intensity to 50% of its initial value for a 60 μl 0.05 mM solution of DPS. These data are summarized in Fig. 3 , which is a graphic comparison of the relative photostabilities of anti -B 18 H 22 and DPS as well as other commercial state-of-the-art blue laser dyes belonging to different families (BBO, Exalite 404, Coumarin 440 and Carbostyril 124, see Supplementary Fig. 2 ) and a batch of colloidal QDs (CdSeS/ZnS core/shell), all of which emit around 400–450 nm. Remarkably, anti -B 18 H 22 presents a photostability that is superior to all but one of the tested laser dyes and even the QDs ( Fig. 3 ). Only Exalite 404, which is the benchmark dye in this spectral region, shows a slightly better photostability than anti -B 18 H 22 . While LIF measurements enable a basis for the absolute comparison of photostability among different dyes, the device lifetime (as a function of the number of pulses) of the actual laser at the point of maximum efficiency is the most relevant figure of merit from a practical point of view. In this regard, the laser efficiency of a small volume (0.5 ml) of a 50 mM cyclohexane solution of anti -B 18 H 22 showed no sign of degradation after 40,000 pulses with a pump energy of 450 μJ at 15 Hz. Only after 80,000 pulses did the efficiency drop to half of the initial value. In terms of time, this translates to 90 min of constant operation per millilitre of solution. The superior resistance to photodegradation of anti -B 18 H 22 with respect to many blue-emitting materials is one of the more remarkable and potentially useful properties of this new kind of laser material. 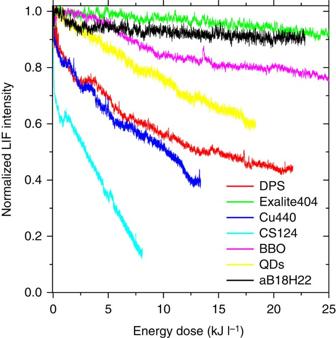Figure 3: Photostability measurements. Plot of laser-induced fluorescence (LIF) intensity normalized to the initial LIF intensity with respect to the absorbed pump energy dose for 60 μl solutions ofanti-B18H22, DPS, Exalite 404, Coumarin 440 (Cu440), Carbostyril 124 (CS124), BBO and CdSeS/ZnS core/shell quantum dots (QDs). (The excitation source was the 3rd harmonic radiation from a Nd:YAG laser. Pulse duration, energy and repetition rate: 20 ns, 0.37 mJ and 15 Hz.) Figure 3: Photostability measurements. Plot of laser-induced fluorescence (LIF) intensity normalized to the initial LIF intensity with respect to the absorbed pump energy dose for 60 μl solutions of anti -B 18 H 22 , DPS, Exalite 404, Coumarin 440 (Cu440), Carbostyril 124 (CS124), BBO and CdSeS/ZnS core/shell quantum dots (QDs). (The excitation source was the 3rd harmonic radiation from a Nd:YAG laser. Pulse duration, energy and repetition rate: 20 ns, 0.37 mJ and 15 Hz.) Full size image Luminescence of anti -B 18 H 22 in polystyrene thin films Regarding commercially available dye lasers, liquid media (dye solutions in organic solvent) are generally preferred, since their fluid nature facilitates cooling via flow systems and guarantees that the gain medium is constantly renewed. However, the use of solution-based lasers do entail a number of inconveniences and limitations, mainly related to the employment and disposal of large volumes of organic solutions (flammable and often carcinogenic), as well as to the technical complexities of the flow systems that are complicated to handle, maintain and clean. The incorporation of laser materials into solid-state matrices mitigates these limitations significantly [29] , [30] . Solid matrices, such as polymers, avoid the use of complex cells or flow systems and after degradation, samples are simply replaced by new ones in a consumable fashion, which in turn enables the use of such lasers by non-highly specialized staff. Another advantage of incorporating chromophores into polymers is that the solid material may be cast as thin films acting as wave-guiding active devices. In fact, there has been significant work over the last few years exploring the development of these types of devices because of their potential applications as coherent light sources suitable for integration in optoelectronic and disposable spectroscopic and sensing devices [30] , [31] , as well as its use as luminescent solar concentrators for energy-harvesting applications [32] . In this regard, the boranes might be a potential candidate, as chromophores in luminescent solar concentrators should have minimal reabsorption (large Stokes shifts), fluorescence quantum yields above 0.90 and high photostabilities [33] , requirements that are fulfilled by the fluorescent boron hydride, anti -B 18 H 22 . Therefore, as a proof-of-concept preliminary experiment to ascertain whether anti -B 18 H 22 could be incorporated into a solid matrix and maintain its fluorescence properties, a chloroform solution mixture of anti -B 18 H 22 and polystyrene was spin-coated onto a quartz substrate to render ~540 nm-thick thin films (see Methods for preparation details). Encouragingly, once these thin films were fully dried, anti -B 18 H 22 seemed to be perfectly dissolved into the polystyrene polymer matrix (no evidence of organic/inorganic phase separation), even at a concentration of 25 mM (0.52 wt% with respect to polymer), and still showed an intense blue fluorescence under ultraviolet lamp irradiation ( Fig. 4 ). This observation, although preliminary, significantly increases the prospects and value of anti -B 18 H 22 , in particular, and boranes, in general, as future photonic materials. 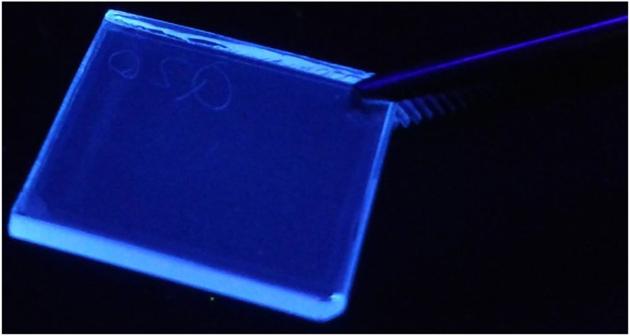Figure 4: Borane in solid matrix. Photograph of polystyrene thin-film doped withanti-B18H2225 mM under ultraviolet irradiation (256 nm). Figure 4: Borane in solid matrix. Photograph of polystyrene thin-film doped with anti -B 18 H 22 25 mM under ultraviolet irradiation (256 nm). Full size image A reasonable extrapolation from the successful incorporation of anti -B 18 H 22 into polystyrene polymer matrices is whether these thin films can sustain stimulated emission and thus permit their development as solid-state integrated lasers. However, using the methods to our disposition, neither amplified spontaneous emission nor laser emission could be excited in these thin films. This is not an indication of low efficiency of the system, but rather a consequence of the low absorption coefficient of the thin film at the pump wavelength ( α ~90 cm −1 ; absorbed light, <1%), which does not allow the system to reach its laser threshold. Therefore, in terms of solid-state laser performance, anti -B 18 H 22 cannot, for the time being, rival other existing solid-state, solution-processable, blue-laser media [34] , [35] , [36] , [37] , [38] . In this regard, further research into the development of new luminescent boranes with stronger absorption properties will ultimately delineate the prospects of efficient and photostable thin-film solid-state borane lasers going forward. In closing, we have demonstrated that solutions of anti -B 18 H 22 function as a blue laser with a good efficiency of 9.5% and an outstanding resistance to photodegradation. Its excellent solubility in organic environments enables the incorporation of anti -B 18 H 22 into polystyrene polymer matrices, without the loss of its fluorescence properties. In addition, theoretical calculations of the laser threshold ( E th ) for solutions of anti -B 18 H 22 suggest considerable scope for the improvement of its laser efficiency. To this end, an increase in the absorbance coefficient of the borane species at the pumping wavelength is desirable, such that lower concentrations could be used for lasing. This would considerably reduce problems of self-quenching, optical scattering and self-absorption losses. It has not escaped our thoughts that perhaps rational modification of the eighteen-vertex borane cluster structure could possibly lead to such desired changes in absorption coefficient, and, in this regard, anti -B 18 H 22 would become the first of a new family of laser materials—the laser boranes. Indeed, very recent and preliminary experimentation in our laboratories reveal that the functionalization of the borane cluster anti -B 18 H 22 (with different functional groups and/or varying number of functional groups) leads to new derivatives that show strong fluorescence at different wavelengths through the visible region. These observations suggest the boranes to be useful compounds to build tunable sources of light emission. Work is currently in progress towards the control of these functionalization processes, and optimization of synthetic and purification protocols. Borane preparation Anti -B 18 H 22 was synthesized by the iodine oxidation of the [B 9 H 12 ] − anion according to the method described in the literature [39] . Pure samples were obtained by repeated crystallizations from hot saturated n -hexane solutions, followed by sublimation under vacuum at 135 °C, and had [11] B and 1 H NMR and mass spectroscopic characteristics in agreement with the published data [21] , [40] . The resulting crystalline powder is readily soluble in organic non-polar aprotic solvents (for example, cyclohexane) and can thus be handled experimentally in an analogous way to that of well-known organic dyes. Therefore, beyond stirring and sonication, no special experimental conditions were necessary for the preparation of laser solutions or for the collection of data, and we could base our study on the vast amount of knowledge on dye laser science and technology in the literature [28] , [41] , [42] . Solution preparation Solutions of anti -B 18 H 22 were prepared in non-polar aprotic solvents, as this compound is otherwise prone to deprotonation (pKa=2.68), which would lead to the formation of its [B 18 H 21 ] − anion and the loss of the compound’s fluorescent emission. Anti -B 18 H 22 exhibits a rather low molar extinction coefficient at the pump wavelength ( ε (at 337 nm) ~5,625 M −1 cm −1 ), which necessitates the use of highly concentrated solutions to achieve the optical densities required in transversal pumping (OD~20). As anti -B 18 H 22 is not soluble in hexane at such concentrations, we used fresh cyclohexane instead. DPS was purchased from Lambdachrome (available currently from Exciton Inc.) and was dissolved in 1,4-dioxane. BBO, Exalite 440 and Coumarin 440 were purchased from Exciton Inc. and dissolved in toluene, p -dioxane and methanol, respectively. Carbostyril 124 and CdSeS/ZnS core/shell QDs were purchased from Aldrich and dissolved (or diluted in the case of QDs), in ethanol and toluene, respectively. The solutions were sonicated and stirred until complete dissolution of compounds, and placed in spectroscopic quartz cuvettes carefully sealed to avoid solvent evaporation. 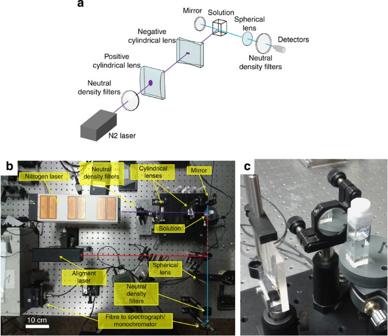Figure 5: Experimental setup for laser measurements. (a) A sketch of the experimental setup. (b) An aerial photograph of the experimental setup for laser measurements. (c) A Close-up view of a photograph of laser cavity. Laser measurements setup Figure 5 shows a sketch and an aerial photograph of the experimental setup used for the laser experiments. The samples were optically pumped at 337.1 nm with 4 ns full-width-at-half-maximum (FWHM) pulses from a nitrogen laser (upgraded MNL-100 from Laser Technik Berlin) operated at 10 or 30 Hz repetition rate. The maximum pump energy reaching the cuvette was 220 μJ. The pump energy was controlled through calibrated neutral-density filters. The light incident on the sample was perpendicular to the surface of the cuvette and focused onto that surface in a stripe shape 1 cm long and 200 μ wide by a combination of negative and positive cylindrical quartz lenses ( f =−15 and +15 cm, respectively), perpendicularly arranged. The oscillation cavity was L 0 =3.5 cm long and had a 90% reflectivity aluminium back mirror together with the end face of the cuvette as the output coupler (4.7% reflectivity). Figure 5: Experimental setup for laser measurements. ( a ) A sketch of the experimental setup. ( b ) An aerial photograph of the experimental setup for laser measurements. ( c ) A Close-up view of a photograph of laser cavity. Full size image The laser emission was collected with a 5 cm focal length spherical lens, focused onto a fibre bundle and detected with a spectrograph/monochromator (Spectrapro-300i Acton Research), equipped with a thermoelectrically cooled charge-coupled device (CCD) detector (SpectruMM:GS 128B) to acquire the spectra, and a photomultiplier (Hamamatsu R928) for the photostability measurements. Calibrated neutral-density filters were used before the fibre bundle to avoid saturation of the detector. For the efficiency measurements, a pyroelectric energy meter (GenTec ED-100A and ED-200) was placed at the exit of the output coupler. Residual pump light was sent into a photodiode acting as the trigger. The trigger signal was fed to a boxcar (Stanford Research, model 250) to convert it to a delayed transistor-transistor logic (TTL) pulse to start the CCD or photomultiplier acquisition. The signal from the CCD was sent directly to a Personal Computer (PC) card, while the signal from the photomultiplier was fed again to the boxcar to be integrated before being digitized and processed by a computer. Alternative laser sources For purposes of experimental thoroughness, we employed two other standard pumping sources in addition to the nitrogen laser, with pumping wavelengths at two positions either side of the peak maximum of the absorption band of anti -B 18 H 22 . Thus, pumping of cyclohexane solutions of anti -B 18 H 22 at 355 nm with the 3rd harmonic of a Nd:YAG (Lotis TII SL-2132, 20 ns FWHM pulses, 15 Hz repetition rate) laser led to observable, but not measureable, laser emission. Pumping with an Xe-Cl excimer laser (Lambda Physik LPX 105i, 20 ns FWHM pulses, 2 Hz repetition rate), emitting at 308 nm, gave a weak laser emission with an efficiency of about 3% ( Supplementary Fig. 3 ). In each case, there was bubble formation in the excited area due to excessive pump energy (~5–10 mJ). In the experiment with the excimer laser, reducing the pump energy to levels at which there was no bubble formation, resulted in output energies too low to be measured. Therefore, in summary, optimal laser efficiency was achieved from pumping with a nitrogen laser at a wavelength 337 nm. Photostability measurements The pumping energy and geometry were exactly equal to that of the laser experiments (see Fig. 5 ). We used spectroscopic quartz cuvettes with 1 cm optical paths and depths L =0.1 cm to allow for the minimum solution volume ( V S =60 μl) to be excited. The lateral facets were grounded, whereupon no laser oscillation was obtained. To avoid stimulated emission processes, and to only monitor the amount of active molecules still available, we used low-concentration solutions in which only LIF was observed. Absorbed energy dose A proper comparison of photostability measurements obtained for different samples and/or materials is a difficult task because of the substantial differences in the experimental conditions, such as pump intensity, pump repetition rate, dye concentration or excited volume. To facilitate comparisons independently of the experimental setup and sample, Dai et al. [43] introduced a normalized photostability defined as the accumulated pump energy absorbed by the system, per litre of solution, before the output energy falls to one-half its initial value. In terms of experimental parameters, this energy dose, in units of kJ l −1 , can be expressed as: where E pump is the energy per pulse in Joules, C is the molar concentration, ε is the molar absorption coefficient in units of M −1 cm −1 , L is the depth of the cuvette expressed in cm, V S is the solution volume, in litres, within the cuvette and f is the ratio between the LIF intensity after #pulses and the LIF intensity in the first pulse. It can be shown that Σ f accounts for the reduction in pump absorption due to species photodegradation. Laser threshold analysis In the theoretical formalism for the threshold pump photon flux ( I pc ) developed by Heudorfer and Marowsky [26] (equation 1) κ is the single-pass loss coefficient that is related to the cavity reflectivities ( R 1 : rear-mirror; R 2 : output coupler) and other non-resonant losses ( α 0 ) such as optical scattering: In addition, p describes the ratio of excited ( L E =1 cm) and unexcited ( L U =2.5 cm) cavity pathlengths ( L E + L U = L 0 ): N tot is the ground-state population density, τ is the fluorescence lifetime, σ ap 0 and σ al 0 are the ground-state absorption cross-sections at the pump and laser wavelengths and σ al 1 is the excited singlet-state absorption cross-section at the laser wavelength. Absorption cross-section ( σ ap 0 ) and molar extinction coefficient ( ε ) are related through the expression: σ ap 0 =ln(10)·1,000· ε / N A , where N A is Avogadro’s number. σ e is the stimulated emission cross-section and is given by σ e =[ λ 4 E ( λ )]/8 πcη 2 τ , where E ( λ ) is the S 1 → S 0 fluorescence spectrum normalized, so that ∫ E ( λ ) dλ = Φ F , Φ F being the fluorescence quantum yield, and η the refractive index of the solution. Preparation of anti -B 18 H 22 /polystyrene thin films A chloroform solution of polystyrene (Mw~192000, Aldrich) (30 mg ml −1 ) mixed with anti -B 18 H 22 (25 mM or 0.52 wt% with respect to polymer) was stirred overnight to ensure complete solution homogeneity. 80 μl aliquots of this solution were then deposited onto clean fused quartz substrates (1 × 1 cm) and immediately spun for 30 s at 1,000 r.p.m. using a spin-coater device before subsequently drying in an oven set at 70 °C to remove residual traces of solvent. The thickness of the resultant thin films, of around 540 nm, was determined by means of interference signatures in the absorption spectra [44] . Such thin films render absorption coefficients (absorbances) for the borane of α ~260 cm −1 (0.006) and α ~90 cm −1 (0.002) at peak (330 nm) and pump (355 nm) wavelengths, respectively. How to cite this article : Cerdán, L. et al. A borane laser. Nat. Commun. 6:5958 doi: 10.1038/ncomms6958 (2015).